Finite-key analysis for measurement-device-independent quantum key distribution Quantum key distribution promises unconditionally secure communications. However, as practical devices tend to deviate from their specifications, the security of some practical systems is no longer valid. In particular, an adversary can exploit imperfect detectors to learn a large part of the secret key, even though the security proof claims otherwise. Recently, a practical approach—measurement-device-independent quantum key distribution—has been proposed to solve this problem. However, so far its security has only been fully proven under the assumption that the legitimate users of the system have unlimited resources. Here we fill this gap and provide a rigorous security proof against general attacks in the finite-key regime. This is obtained by applying large deviation theory, specifically the Chernoff bound, to perform parameter estimation. For the first time we demonstrate the feasibility of long-distance implementations of measurement-device-independent quantum key distribution within a reasonable time frame of signal transmission. It is unequivocal that quantum key distribution (QKD) [1] , [2] needs to bridge the gap between theory and practice. In theory, QKD offers perfect security. In practice, however, it does not, as most practical devices behave differently from the theoretical models assumed in the security proofs. As a result, we face implementation loopholes, or so-called side channels, which may be used by adversaries without being detected, as seen in recent attacks against certain commercial QKD systems [3] , [4] , [5] , [6] , [7] , [8] , [9] , [10] , [11] . There are two potential ways to guarantee security in the realization of QKD. The first is to develop mathematical models that perfectly match the behaviour of physical apparatuses, and then incorporate this information into a new security proof. While this is plausible in theory, unfortunately it is very hard to realize in practice, if not impossible. The second alternative is to design new protocols and develop security proof techniques that are compatible with a wide class of device imperfections. This allows us to omit an accurate characterization of real apparatuses. The most well-known example of such a solution is (full) device-independent QKD (diQKD) [12] , [13] , [14] , [15] , [16] . Here the legitimate users of the system (typically called Alice and Bob) treat their devices as two quasi ‘black boxes’—that is, they need to know which elements their boxes contain, but not how they fully function [17] . The security of diQKD relies on the violation of a Bell inequality [18] , [19] , which certifies the presence of quantum correlations. Despite its beauty, however, this approach is highly impractical because it requires a loophole-free Bell test that at the moment is still unavailable [20] . Also, its secret key rate at practical distances is very limited [21] , [22] . Very recently, a novel approach has been introduced, which is fully practical and feasible to implement. This scheme is known as measurement-device-independent QKD (mdiQKD) [23] and offers a clear avenue to bridge the gap between theory and practice. Its feasibility has been promptly demonstrated both in laboratories and via field tests [24] , [25] , [26] , [27] . It successfully removes all (existing and yet to be discovered) detector side channels [3] , [5] , [6] , [9] , [10] , [11] , which, arguably, is the most critical part of most QKD implementations. Importantly, in contrast to diQKD, this solution does not require that Alice and Bob perform a loophole-free Bell test; it is enough if they prove the presence of entanglement in a quantum state that is effectively distributed between them, just like in standard QKD schemes [28] . In addition, now Alice and Bob may treat the measurement apparatus as a true ‘black box’, which may be fully controlled by the adversary. A slight drawback is that Alice and Bob need to characterize the quantum states (for example, the polarization degrees of freedom of phase-randomized weak coherent pulses (WCPs)) that they send through the channel. However, as this process can be verified in a protected environment outside the influence of the adversary, it is less likely to be a problem. For completeness, the readers can refer to ref. 29 where a characterization of the prepared states is no longer required. Nevertheless, so far the security of mdiQKD has only been proven in the asymptotic regime [23] , which assumes that Alice and Bob have access to an unlimited amount of resources, or in the finite regime but only against particular types of attacks [30] , [31] . In summary, until now, a rigorous security proof of mdiQKD that takes full account of the finite size effects [32] , [33] , [34] has appeared to be missing and, for this reason, the feasibility of long-distance implementations of mdiQKD within a reasonable time frame of signal transmission has remained undemonstrated. The main contributions of this work are twofold. First, in contrast to existing heuristic results on mdiQKD, we provide, for the first time, a security proof in the finite-key regime that is valid against general attacks and satisfies the composability definition [35] , [36] of QKD. Second, we apply large deviation theory, specifically a multiplicative form of the Chernoff bound [37] , to perform the parameter estimation step. The latter is crucial to demonstrate that a long-distance implementation of mdiQKD (for example, 150 km of optical fibre with 0.2 dB km −1 ) is feasible within a reasonable time frame. To obtain high secret key rates in this scenario, it is common to use decoy state techniques [38] , [39] , [40] , both for standard QKD protocols and mdiQKD. Here a key challenge is to estimate the transmittance and the quantum bit error rate (QBER) of the single-photon component of the signal at the presence of high losses (for example, 30 dB). We show that such an estimation problem can be solved using the Chernoff bound, as it provides good bounds for the above parameters even in the high-loss regime. We highlight that our results can be applied to other QKD protocols (for example, the standard decoy state BB84 protocol [38] , [39] , [40] ) as well as to general experiments in quantum information. Security definition Before stating the protocol, let us quickly review the security framework [35] , [36] that we are considering here. A general QKD protocol (executed by Alice and Bob) generates either a pair of bit strings S A and S B , or a symbol to indicate the abort of the protocol. In general, the string of Alice, S A , can be quantum mechanically correlated with a quantum state that is held by the adversary. Mathematically, this situation is described by the classical quantum state where denotes an orthonormal basis for Alice’s system, and the subscript E indicates the system of the adversary. Ideally, we say that a QKD protocol is secure if it satisfies two conditions, namely the correctness and the secrecy. The correctness condition is met if S A = S B , that is, Alice’s and Bob’s bit strings are identical. The secrecy condition is met if , where is the uniform mixture of all possible values of the bit string S A . That is, the system of the adversary is completely decoupled from that of Alice. Owing to the presence of errors, however, these two conditions can never be perfectly met. For example, in the finite-key regime it is impossible to guarantee S A = S B with certainty. In practice, this implies that we need to allow for some minuscule errors. That is, we say that a QKD scheme is ε cor -correct if , that is, the probability that Alice’s and Bob’s bit strings are not identical is not greater than ε cor . Similarly, we say that a protocol is, ε sec -secret if where denotes the trace norm. That is, the state ρ AB is ε sec -close to the ideal situation described by . Thereby a QKD protocol is said to be ε -secure if it is both ε cor -correct and ε sec -secret, with . With this security definition we are able to guarantee that the security of the protocol holds even when combined with other protocols, that is, the protocol is secure in the so-called universally composable framework [35] , [36] . Protocol definition The set-up is illustrated in Fig. 1 . Alice and Bob use a laser source to generate quantum signals that are diagonal in the Fock basis. Instances of such sources include attenuated laser diodes emitting phase-randomized WCPs, triggered spontaneous parametric downconversion sources and practical single-photon sources. Each pulse is prepared in a different BB84 state [41] , which is selected, for example, uniformly at random from two mutually unbiased bases, denoted as Z and X. The signals are then sent to an untrusted relay Charles, who is supposed to perform a Bell state measurement that projects them into a Bell state. Also, Alice and Bob apply decoy state techniques [38] , [39] , [40] to estimate the gain (that is, the probability that the relay outputs a successful result) and the QBER for various input photon numbers. 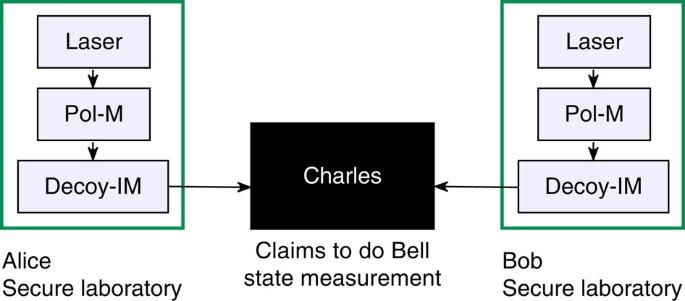Figure 1: A schematic diagram of mdiQKD. Alice and Bob prepare quantum signals in different BB84 polarization states41with a polarization modulator (Pol-M). Also, they use an intensity modulator (Decoy-IM) to generate decoy states. The signals are sent to an untrusted relay Charles, who is supposed to perform a Bell state measurement that projects the incoming signals into a Bell state. See the main text for details. Figure 1: A schematic diagram of mdiQKD. Alice and Bob prepare quantum signals in different BB84 polarization states [41] with a polarization modulator (Pol-M). Also, they use an intensity modulator (Decoy-IM) to generate decoy states. The signals are sent to an untrusted relay Charles, who is supposed to perform a Bell state measurement that projects the incoming signals into a Bell state. See the main text for details. Full size image Next, Charles announces whether or not his measurements are successful, including the Bell states obtained. Alice and Bob keep the data that correspond to these instances and discard the rest. Also, they post-select the events where they employ the same basis. Finally, either Alice or Bob flips part of her/his bits to correctly correlate them with those of the other. See Box 1 for a detailed description of the different steps of the protocol. Since Charles’ measurement is basically used to post-select entanglement between Alice and Bob, the security of mdiQKD can be proven by using the idea of time reversal. Indeed, mdiQKD builds on the earlier proposals of time-reversed EPR protocols by Biham et al . [42] and Inamori [43] , and combine them with the decoy state technique. The end result is the best of both worlds—high performance and high security. We note on passing that the idea of time reversal has also been previously used in other quantum information protocols including one-way quantum computation. Table 1 Post-processing of data in the sifting step. Full size table Box 1: Protocol definition. State preparation : Alice and Bob repeat the first four steps of the protocol for i =1,…, N until the conditions in the Sifting step are met. For each i , Alice chooses an intensity , a basis , and a random bit with probability p a ,α /2. Here is the intensity of the signal (decoy) states. Next, she generates a quantum signal (for example, a phase-randomized WCP) of intensity a prepared in the basis state of α given by r . Likewise, Bob does the same. Distribution : Alice and Bob send their states to Charles via the quantum channel. Measurement : If Charles is honest, he measures the signals received with a Bell state measurement. In any case, he informs Alice and Bob (via a public channel) of whether or not his measurement was successful. If successful, he reveals the Bell state obtained. Sifting : If Charles reports a successful result, Alice and Bob broadcast (via an authenticated channel) their intensity and basis settings. For each Bell state k , we define two groups of sets: and . The first (second) one identifies signals where Charles declared the Bell state k and Alice and Bob selected the intensities a and b and the basis Z (X). The protocol repeats these steps until and . Next, say Bob flips part of his bits to correctly correlate them with those of Alice (see Table 1 ). Afterwards, they execute the last steps of the protocol for each k . Parameter estimation : Alice and Bob use n k random bits from to form the code bit strings Z k and , respectively. The remaining R k bits from are used to compute the error rate , where are Bob’s bits. If , Alice and Bob assign an empty string to S k and abort steps 6 and 7 for this k . The protocol only aborts if . If , Alice and Bob use and to estimate n k ,0 , n k ,1 and e k ,1 . The parameter n k ,0 , ( n k ,1 ) is a lower bound for the number of bits in Z k where Alice (Alice and Bob) sent a vacuum (single-photon) state. e k ,1 is an upper bound for the single-photon phase error rate. If e k ,1 > e tol , an empty string is assigned to S k and steps 6 and 7 are aborted for this k , and the protocol only aborts if . Error correction : For those k that passed the parameter estimation step, Bob obtains an estimate of Z k using an information reconciliation scheme. For this, Alice sends him leak EC , k bits of error correction data. Next, Alice computes a hash of Z k of length using a random universal 2 hash function, which she sends to Bob together with the hash [35] . If , Alice and Bob assign an empty string to S k and abort step 7 for this k . The protocol only aborts if . Privacy amplification : If k passed the error correction step, Alice and Bob apply a random universal 2 hash function to Z k and to extract two shorter strings of length (see ref. 35 ). Alice obtains S k and Bob . The concatenation of form the secret key S A ( S B ). Security analysis We now present one main result of our paper. It states that the protocol introduced above is both ε cor -correct and ε sec -secret, given that the length of the secret key S A is selected appropriately for a given set of observed values. See Box 1 for the definition of the different parameters that we consider in this section. The correctness of the protocol is guaranteed by its error correction step, where, for each possible Bell state k , Alice sends a hash of Z k to Bob, who compares it with the hash of . If both hash values are equal, the protocol gives except with error probability ε cor /4. If , its output is an empty string (that is, the protocol is trivially correct). Moreover, if the protocol aborts, the result is , that is, it is also correct. This guarantees that S A = S B except with error probability ≤ ε cor . Alternatively to this method, Alice and Bob may also guarantee the correctness of the protocol by exploiting properties of the error-correcting code employed [44] . If the length of each bit string S k , which forms the secret key S A , satisfies the protocol is ε sec -secret, with and . In equation (1), is the binary Shannon entropy, and the parameters ε k ,0 , ε k ,1 , and ε k , e quantify, respectively, the probability that the estimation of the terms n k ,0 , n k ,1 and e k ,1 is incorrect. A sketch of the proof of equation (1) can be found in the Methods section. Also explained there, is the meaning of all the epsilons contained in the term , which we omit here for simplicity. In the asymptotic limit of very large data blocks, the terms reducing the length of S A due to statistical fluctuations may be neglected, and thus satisfies , as previously obtained in ref. 23 . That is, n k ,0 and n k ,1 provide a positive contribution to the secret key rate, while n k ,1 h ( e k ,1 ) and leak EC, k reduce it. The term n k ,1 h ( e k ,1 ) corresponds to the information removed from Z k in the privacy amplification step of the protocol, while leak EC, k is the information revealed by Alice in the error correction step. The second main contribution of this work is an estimation method to obtain the relevant parameters n k ,0 , n k ,1 and e k ,1 needed to evaluate the key rate formula above, when Alice and Bob send Charles a finite number, N , of signals and use a finite number of decoy states. We solve this problem using techniques in large deviation theory. More specifically, we employ the Chernoff bound [37] . It is important to note that standard techniques such as Azuma’s inequality [45] do not give very good bounds here. This is because this result does not consider the properties of the a priori distribution. Therefore, it is far from optimal for situations such as high loss or a highly bias coin flip, which are relevant in long-distance QKD. In contrast, the Chernoff bound takes advantage of the property of the distribution and provides good bounds even in a high-loss regime. More precisely, we show that the estimation of n k ,0 , n k ,1 and e k ,1 can be formulated as a linear program, which can be solved efficiently in polynomial time and gives the exact optimum even for large dimensions [46] . Importantly, this general method is valid for any finite number of decoy states used by Alice and Bob, and for any photon-number distribution of their signals. Also, for the typical scenario where Alice and Bob send phase-randomized WCPs together with two decoy states each, we solve analytically the linear program, and obtain analytical expressions for the parameters above, which can be used directly in an experiment. A sketch of the estimation technique is given in the Methods section. For a detailed analysis of both estimation techniques we refer to the Supplementary Notes 1 and 2 . In this section, we analyse the behaviour of the secret key rate provided in equation (1). In our simulation, we consider that Alice and Bob encode their bits in the polarization degrees of freedom of phase-randomized WCPs. Also, we assume that Charles uses the linear optics quantum relay illustrated in Fig. 2 , which is able to identify two of the four Bell states. With this set-up, a successful Bell state measurement corresponds to the observation of precisely two detectors (associated to orthogonal polarizations) being triggered. Note, however, that the results presented in this paper can be applied to other types of coding schemes like, for instance, phase or time-bin coding [1] , [2] , and to any quantum operation that Charles may perform, as they solely depend on the measurement results that he announces. 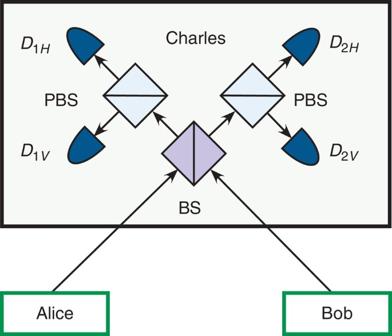Figure 2: A schematic diagram of Charles’ measurement device. The signals from Alice and Bob interfere at a 50:50 beam splitter (BS), which has on each end a polarizing beam splitter (PBS) that projects the incoming photons into either horizontal (H) or vertical (V) polarization states. A click in the single-photon detectorsD1HandD2V, or inD1VandD2H, indicates a projection into the Bell state, while a click inD1HandD1V, or inD2HandD2V, implies a projection into the Bell state Figure 2: A schematic diagram of Charles’ measurement device. The signals from Alice and Bob interfere at a 50:50 beam splitter (BS), which has on each end a polarizing beam splitter (PBS) that projects the incoming photons into either horizontal ( H ) or vertical ( V ) polarization states. A click in the single-photon detectors D 1 H and D 2 V , or in D 1 V and D 2 H , indicates a projection into the Bell state , while a click in D 1 H and D 1V , or in D 2 H and D 2 V , implies a projection into the Bell state Full size image We use experimental parameters from ref. 47 . But, whereas ref. 47 considers a free-space channel, we assume a fibre-based channel with a loss of 0.2 dB km −1 . The detection efficiency of the relay (that is, the transmittance of its optical components together with the efficiency of its detectors) is 14.5% and the background count rate is 6.02 × 10 −6 . Moreover, we use a rather generic channel model that includes an intrinsic error rate that simulates the misalignment and instability of the optical system. This is done by placing a unitary rotation in both input arms of the 50:50 beam splitter, and another unitary rotation in one of its output arms [48] . In addition, we fix the security bound to ε =10 −10 . The results are shown in Figs 3 and 4 for the situation where Alice and Bob use two decoy states each. In this scenario, we obtain the parameters n k ,0 , n k ,1 and e k ,1 using the analytical estimation procedure introduced above (see Supplementary Note 1 for more details). The first figure illustrates the secret key rate (per pulse) as a function of the distance between Alice and Bob for different values of the total number of signals N sent. We fix ε cor =10 −15 ; this corresponds to a realistic hash tag size in practice [35] . Also, we fix the intensity of the weakest decoy states to , since, in practice, it is difficult to generate a vacuum state due to imperfect extinction. This value for and can be easily achieved with a standard intensity modulator. Moreover, for simplicity, we assume an error correction leakage that is a fixed fraction of the sifted key length n k , that is, , with ζ =1.16 and where h (·) is again the binary Shannon entropy [32] . In a realistic scenario, however, the value of ζ typically depends on the value of n k , and when n k <10 5 the parameter ζ may be bigger than 1.16. For a given distance, we optimize numerically over all the free parameters of the protocol. This includes the intensities and , the probability distributions and in the state preparation step, the parameters and in the sifting step, the term n k in the parameter estimation step and the different epsilons contained in ε sec . Our simulation result shows clearly that mdiQKD is feasible with current technology and does not require high-efficiency detectors for its implementation. If Alice and Bob use laser diodes operating at 1 GHz repetition rate, and each of them sends N =10 13 signals, we find, for instance, that they can distribute a 1-Mb secret key over a 75-km fibre link in <3 h. This scenario corresponds to the red line shown in Fig. 3 . Notice that, at telecom wavelengths, standard InGaAs detectors have modest detection efficiency of about 15%. Since mdiQKD requires twofold coincidence rather than single detection events, as is the case in the standard decoy state protocol, the key rate of mdiQKD is lower than that of the standard decoy state scheme. However, with high-efficiency detectors such as silicon detectors [49] in 800 nm or high-efficiency superconducting nanowire single-photon detectors [50] , the key rate of mdiQKD can be made comparable to that of the standard decoy state protocol. 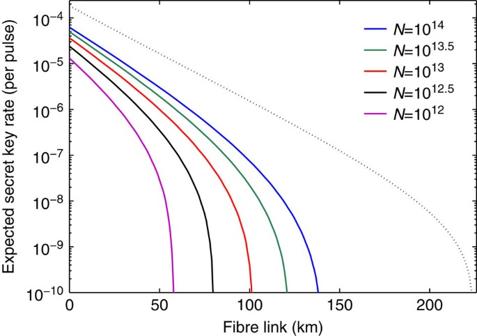Figure 3: Expected key rate as function of the distance. Secret key ratein logarithmic scale for the protocol introduced in the Results section with phase-randomized WCPs as a function of the distance. The solid lines correspond to different values for the total number of signalsNsent by Alice and Bob. The overall misalignment in the channel is 1.5%, and the security boundε=10−10. For simulation purposes we consider the following experimental parameters47: the loss coefficient of the channel is 0.2 dB km−1, the detection efficiency of the relay is 14.5% and the background count rate is 6.02 × 10−6. Our results show clearly that even with a realistic finite size of data, sayN=1012to 1014, it is possible to achieve secure mdiQKD at long distances. In comparison, the dotted line represents a lower bound on the secret key rate for the asymptotic case where Alice and Bob send Charles infinite signals and use an infinite number of decoy settings. Figure 3: Expected key rate as function of the distance. Secret key rate in logarithmic scale for the protocol introduced in the Results section with phase-randomized WCPs as a function of the distance. The solid lines correspond to different values for the total number of signals N sent by Alice and Bob. The overall misalignment in the channel is 1.5%, and the security bound ε =10 −10 . For simulation purposes we consider the following experimental parameters [47] : the loss coefficient of the channel is 0.2 dB km −1 , the detection efficiency of the relay is 14.5% and the background count rate is 6.02 × 10 −6 . Our results show clearly that even with a realistic finite size of data, say N =10 12 to 10 14 , it is possible to achieve secure mdiQKD at long distances. In comparison, the dotted line represents a lower bound on the secret key rate for the asymptotic case where Alice and Bob send Charles infinite signals and use an infinite number of decoy settings. 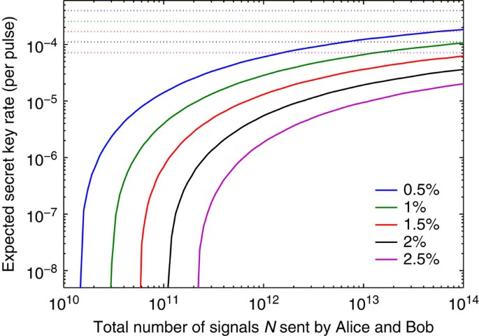Figure 4: Expected key rate as function of the block size. The plot shows the secret key ratein logarithmic scale as a function of the total number of signalsNsent by Alice and Bob in the limit of zero distance. The security boundε=10−10. The solid lines correspond to different values for the intrinsic error rate due to the misalignment and instability of the optical system. The horizontal dotted lines show the asymptotic rates. The experimental parameters are the ones described in the caption ofFig. 3. Our results show that, even for a finite size of signals sent by Alice and Bob, mdiQKD is robust to intrinsic errors due to basis misalignment and instability of the optical system. Full size image Figure 4: Expected key rate as function of the block size. The plot shows the secret key rate in logarithmic scale as a function of the total number of signals N sent by Alice and Bob in the limit of zero distance. The security bound ε =10 −10 . The solid lines correspond to different values for the intrinsic error rate due to the misalignment and instability of the optical system. The horizontal dotted lines show the asymptotic rates. The experimental parameters are the ones described in the caption of Fig. 3 . Our results show that, even for a finite size of signals sent by Alice and Bob, mdiQKD is robust to intrinsic errors due to basis misalignment and instability of the optical system. Full size image The second figure illustrates as a function of N for different values of the misalignment in the limit of zero distance. For comparison, this figure also includes the asymptotic secret key rate when Alice and Bob send an infinite number of signals and use an infinite number of decoy states [23] . Our results show that significant secret key rates are already possible with 10 11 signals, given that the error rate is not too large. In conclusion, we have proved the security of mdiQKD in the finite-key regime against general attacks. This is the only known fully practical QKD protocol that offers an avenue to bridge the gap between theory and practice in QKD implementations. Importantly, our results clearly demonstrate that even with practical signals (for example, phase-randomized WCPs) and a finite size of data (say 10 12 to 10 14 signals) it is possible to perform secure mdiQKD over long distances (up to about 150 km). To achieve high secret key rates in such high-loss regime, it is typical for both standard QKD schemes and mdiQKD to use decoy state techniques. A main challenge in this scenario is to obtain tight bounds for the gain and QBER of the single-photon components sent by Alice and Bob. We have shown that this estimation problem can be successfully solved using techniques in large deviation theory, more precisely, the Chernoff bound. This result takes advantage of the property of the distribution, and thus provides good bounds for the relevant parameters even in the presence of high losses, as is the case in QKD realizations. Using the Chernoff bound, we have rewritten the problem of estimating the gain and QBER of the single-photon signals as a linear program, which can be solved efficiently in polynomial time. This general method is valid for any finite number of decoy states, and for any photon-number distribution of the signals. It can be used, for instance, with laser diodes emitting phase-randomized WCPs, triggered spontaneous parametric downconversion sources and practical single-photon sources. Also, for the common scenario where Alice and Bob send phase-randomized WCPs together with two decoy states each, we have obtained tight analytical bounds for the quantities above. These results apply to different types of coding schemes like, for example, polarization, phase or time-bin coding. Secrecy Here we briefly discuss on the secrecy of the protocol described in Box 1 . To begin with, note that Alice and Bob obtain the error rate using a random sample of of size R k . This means that when satisfies the tolerated value E tol , the error rate between the strings Z k and , which we denote as , satisfies the following inequality written as conditional probability [51] where . Here the parameter Ω pass represents the event that all the tests performed during the realization of the protocol satisfy the tolerated values. Let denote the adversary’s information about Z k up to the error correction step in Box 1 . By using a privacy amplification scheme based on two-universal hashing [35] we can generate an ε k -secret string S k of length , where ε k >0, and The function denotes the smooth min-entropy [35] , [52] . It quantifies the average probability that the adversary guesses Z k correctly using the optimal strategy with access to . The term can be decomposed as , where C k is the information revealed by Alice and Bob during the error correction step, and E k is the adversary’s information before that step. Using a chain rule for smooth entropies [35] , we obtain with . The bits of Z k can be distributed among three different strings: . The first contains bits where Alice sent a vacuum state, the second where both Alice and Bob sent a single-photon state and includes the rest of bits. Using the result from ref. 53 , we have that where . Here we have used the fact that , and . The latter arises because vacuum states contain no information about their bit values, which are uniformly distributed. The next step is to obtain a lower bound for the term . Taking that Alice and Bob do the state preparation scheme perfectly in the Z and X bases (that is, they prepare perfect BB84 states), we can re-write this quantity in terms of the smooth max-entropy between them, which is directly bounded by the strength of their correlations [32] . More precisely, the entropic uncertainty relation gives us Combining equations (3)–(6), we find that a secret key of length given by equation (1) gives an error of . Finally, after composing the errors related with the estimation of n k ,0 , n k ,1 and e k ,1 , selecting and equal to zero, and also removing the conditioning on Ω pass , we obtain a security parameter given by where , and ε k ,0 , ε k ,1 and ε k , e , denote, respectively, the error probability in the estimation of n k ,0 , n k ,1 and e k ,1 . Parameter estimation To simplify the discussion, let us consider the estimation of the parameter n k ,0 . The method to obtain n k ,1 and e k ,1 follows similar arguments. The procedure can be divided into two steps. First, we calculate a lower bound for the number of indexes in where Alice sent a vacuum state. This quantity is denoted as m k ,0 . Second, we compute n k ,0 from m k ,0 using the Serfling inequality for random sampling without replacement [51] . In the first step we use a multiplicative form of the Chernoff bound [37] for independent random variables, which does not require the prior knowledge on the population mean. More precisely, we use the following claim. Claim: Let , be a set of independent Bernoulli random variables that satisfy Pr( X i =1)= p i , and let and , where E [·] denotes the mean value. Let x be the observed outcome of X for a given trial (that is, ) and for certain . When and for a certain , we have that x satisfies except with the error probability , where the parameter , with , and . Here denotes the probability that . Importantly, the bounds (−Δ and ) on the fluctuation parameter δ that appears in equation (8) do not depend on the mean value μ . A proof of this claim can be found in the Supplementary Note 3 . There we introduce as well a generalized version of the claim for the cases where and/or . To apply this statement and be able to obtain the parameter m k ,0 , we rephrase the protocol described in Box 1 . For each signal, we consider that Alice (Bob) first chooses a photon-number n ( m ) and sends the signal to Charles, who declares whether his measurement is successful or not. After Alice decides the intensity setting a , Bob does the same. This virtual protocol is equivalent to the original one because the essence of decoy state QKD is precisely that Alice and Bob could have postponed the choice of which states are signals or decoys after Charles’ declaration of the successful events. This is possible because Alice’s and Bob’s observables commute with those of Charles. Note that for each specific combination of values n and m , the observables that Alice and Bob use to determine whether a state is a signal or a decoy act on entirely different physical systems from those of Charles. This implies that Alice and Bob are free to postpone their measurement and thus their choice of signals and decoys. Also, this result shows that for each combination n and m , the signal and decoy states provide a random sample of the population of all signals containing n and m photons, respectively. Therefore, one can apply random sampling theory in classical statistics to the quantum problem. Let denote the set that identifies those signals sent by Alice and Bob with n and m photons, respectively, when they select the Z basis and Charles announces the Bell state k . And, let , and be the conditional probability that Alice and Bob have selected the intensity settings a and b , given that their signals contain, respectively, n and m photons prepared in the Z basis. Then, if we apply the above equivalence, independently of each other and for each signal Alice and Bob assign to each element in the intensity setting a , b , with probability . Let be if the i th element of is assigned to the intensity setting combination a , b , and otherwise 0. And, let with . Let denote the observed outcome of the random variable for a given trial. Then, if and , with the Claim above implies that except with error probability , where , with and . Using similar arguments, we find that the parameter m k ,0 can be written as except with error probability ε 0 , where . Now it is easy to find a lower bound for m k ,0 . One only needs to minimize equation (12) given the linear constraints imposed by equation (11) for all a , b . This problem can be solved either by using numerical tools as linear programming [46] or, for some particular cases, by using analytical techniques. See Supplementary Notes 1 and 2 for details. The second step of the procedure is quite direct. Note that Alice forms her bit string Z k using n k random indexes from . Using ref. 51 we obtain except with error probability where corresponds to the total error probability in the estimation of , and the function is defined as . How to cite this article: Curty, M. et al . Finite-key analysis for measurement-device-independent quantum key distribution. Nat. Commun. 5:3732 doi: 10.1038/ncomms4732 (2014).